G-protein β2 subunit interacts with mitofusin 1 to regulate mitochondrial fusion Mitofusins (Mfns) mediate the fusion of mitochondrial membranes. However, little is known about how Mfns are regulated to control mitochondrial fusion, which is a multistep process requiring tethering and docking of the outer membranes of two mitochondria. In this study, we report that guanine nucleotide binding protein-β subunit 2 (Gβ2), a WD40 repeats protein and a member of the β-subunits of the heterotrimeric G proteins, has a crucial function in mitochondrial fusion. Gβ2 was found to be enriched on the surface of mitochondria and interacted with mitofusin 1 (Mfn1) specifically. Gβ2 also regulated the mobility of Mfn1 on the surface of the mitochondrial membrane and affected the mitochondrial fusion. Depletion of endogenous Gβ2 resulted in mitochondrial fragmentation, which could be rescued by exogenous Gβ2. These findings have thus uncovered a novel role of Gβ2 in regulating mitochondrial fusion through its interaction with Mfn1. Mitochondria are dynamic organelles undergoing constant fusion and fission, and dysregulation of mitochondrial dynamics has been linked to altered mitochondrial physiology, abnormal mitochondrial DNA maintenance, apoptosis [1] , [2] and neuromuscular diseases [3] , [4] . These two opposing processes are regulated by two members of the dynamin family: mitofusins (Mfns) and dynamin-related guanosine triphosphatases (GTPases) (Drp1) [5] , [6] . Proper control of mitochondrial fission and fusion is vital to both the integrity of the mitochondrial morphology and their functions [7] , [8] , [9] , [10] , [11] . Several WD40 proteins, such as Mdv1 and Caf4, are found to interact with Dnm1, a major mediator for mitochondrial fission in yeast, to determine the localization of Dnm1 on the mitochondrial surface [12] and modulate the process of fission, at least in the yeast system [13] . Mfn 1/2, two mitochondrial GTPases in the dynamin family, mediate the fusion of mitochondrial membrane. During these processes, Mfn1 and Mfn2 act in a trans -manner leading to a closer apposition of the membranes for completing the fusion [14] . Removal of the GTPase domain of Mfn1 is still able to induce the aggregation of mitochondria without complete fusion [14] , [15] , suggesting that domains other than GTPase activity are required for mitochondrial docking or tethering. We reasoned that there may be other factors that act to coordinate Mfns for mitochondrial fusion. In this study, we report that guanine nucleotide binding protein-β subunit 2 (Gβ2), a member of the β-subunits of the heterotrimeric G proteins and a WD40 protein, has a crucial function for mitochondrial fusion. Gβ2 is partially found on the surface of mitochondria and physically interacts with Mfn1. Depletion of Gβ2 perturbs mitochondrial morphology and decrease mitochondrial fusion rate. Gβ2 acts by limiting the membrane mobility of Mfn1 at the mitochondrial surface to regulate the process of mitochondrial fusion. These findings demonstrated that Gβ2 interacts with mfn1 to regulate mitochondrial fusion. Gβ2 localizes to the surface of mitochondria To identify potential proteins regulating Mfns, we used a yeast two hybrid assay to identify potential molecules, which may interact with Mfn 1 or 2 by using the full-length Mfn1 and Mfn 2, or different domains of Mfn1 as baits. As a result, we obtained 91 positive clones, 3 of which encoded Gβ2 when the fragment of aa241–387 was used as a bait. Gβ2 interaction with Mfn1 is specific, as reconstitution of AD (active domain)-Gβ2 (in the fish vector) with BD (binding domain)-Mfn1 (in the bait vector), but not with BD-Mfn2, gave a strong positive result (see Supplementary Fig. S1a ). Structural analysis has revealed that the Gβ subunits are WD40 repeat proteins with a toroidal structure containing seven-bladed β-propellers [16] . The unique toriodal β-propeller structure defines surfaces for interactions with numerous receptors, Gα and many other effectors [17] . Despite accumulating evidence that has shown Gβγ dimers exert its functions on various effectors as the Gα proteins do [18] , [19] , [20] , the role of Gβ2 in mitochondrial dynamics is largely unknown. Thus, we first examined if Gβ2 and Mfns are co-localized in mitochondria by immunostaining. Indeed, our data revealed that endogenous Gβ2 was localized in mitochondria in HeLa ( Fig. 1a ) and SH-SY5Y neuroblastoma cells ( Supplementary Fig. S1b ). In contrast, a specific antibody to Gβ1, most similar to Gβ2 in amino acids identity among all Gβ subunits, showed diffused staining in HeLa cells ( Fig. 1b ). Confocal microscopic analysis showed that Gβ2 appeared to have a patchy distribution along the mitochondrial tubular structure, and this observation was substantiated by three-dimensional analysis using the scanned confocal images ( Fig. 1a ). To further ascertain that Gβ2 is indeed localized in mitochondria, we performed a gradient fractionation assay. HeLa cells were homogenized with a Dounce homogenizer and the cell lysates were separated into the crude mitochondrial fraction, 10,000× g supernatant (C 2 ) containing plasma membrane, the microsomal fraction, as well as cytosolic proteins. The crude mitochondrial fraction and C 2 were further fractionated by Percoll density gradient centrifugation to obtain pure mitochondrial fraction (M), plasma membrane fraction (P) and the cytosol (C 1 ). The purity of the mitochondrial fractions was tested by loading equal amount of proteins onto a gel validated by using mitochondrial-specific markers such as VDAC1 and Mfn1, and by specific markers for endoplasmic reticulum (p62 (ref. 21 )), Golgi (GM130 (ref. 22 )). 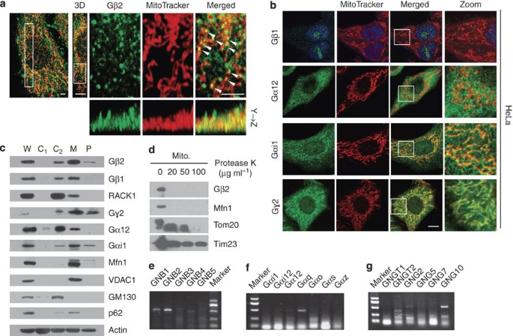Figure 1: Distribution of Gβ2 protein on the surface of mitochondria. (a) Immunostaining with a specific antibody shows the localization of Gβ2 in HeLa cells. Cells were stained with 20 nM Mitotracker Red, and then immuno-labelled with anti-Gβ2 (green) and visualized with a two-photon microscope (Zeiss, LSM 510). The boxed area on the upper left was scanned along the Z axis, and the images were superposed to form the three-dimensional (3D) image. The boxed area in the 3D image is shown at higher magnification in the upper right panels. The lower right shows images of Y to Z dimension. Scale bar, 20 μm. (b) Distribution of Gβ1, Gα12, Gαi1 and Gγ2 in HeLa cells. Representative images of HeLa cells labelled with anti-Gβ1, Gα12, Gαi1 and Gγ2 antibodies (green) and stained with 20 nM Mitotracker Red. Scale bar, 10 μm. (c) Distribution of Gβ2 and other G proteins in the mitochondrial fraction. Equal amounts of the whole cell lysate (W), cytosol (C1), light membrane (C2), mitochondria (M) and plasma membrane (P) fractions were loaded and analysed for the distribution of Gβ2, Gγ2 and other G proteins by western blot using specific antibodies. The purity of isolated mitochondria was determined by using the markers for distinct organelles: Mfn1, VDAC1 (mitochondria), GM130 (Golgi), p62 (endoplasmic reticulum) and actin (cytoplasm). (d) Protease K assay for Gβ2's localization on mitochondria. Mitochondrial fractionation obtained from HeLa cells was subjected to Protease K digestion for 30 min with different concentrations as indicated. Gβ2 and other mitochondrial proteins such as Mfn1, Tom20 (outer mitochondrial membrane, OMM) and Tim23 (inner mitochondrial membrane, IMM) were analysed by western blot with corresponding antibodies. Equal amounts of protein were loaded for Protease K treatment. (e) Gβ2 is the most abundant subunit of Gβ proteins in HeLa cells. mRNA levels of distinct Gβ subunits were analysed by semiquantitative PCR in HeLa cells. (f,g) The mRNA levels of Gα, Gγ subunits in the cells were analysed by semiquantitative PCR (right panel). The size markers are 1,000, 750, 500, 200 and 100 bp, respectively, from top to bottom. All the experiments were repeated at least three times. As shown in Figure 1c , Gβ2, but not Gβ1, was significantly enriched in the purified mitochondrial fraction compared with other fractions (enrichment 48.5%). Gγ2 was also enriched in the purified mitochondrial fraction, whereas Gγ1 was not detectable. Gα12 and Gαi1 were present in mitochondria, which were consistent with previous reports [23] , [24] , and other membrane fractions. To determine the precise localization of Gβ2 on the outer membrane, we incubated intact mitochondria isolated from HeLa cells with protease K. Our data showed that Gβ2, similar to Tom20 and Mfn1 that are mitochondrial outer membrane proteins, was sensitive to protease K ( Fig. 1d ). Furthermore, Gβ2 was resistant to NaHCO 3 treatment, suggesting that Gβ2 does not adhere to the outer membrane of the mitochondria nonspecifically [25] . Semiquantitative PCR analysis showed that Gβ2 is expressed at high levels in both HeLa and SH-SY5Y cells ( Fig. 1e–g , Supplementary Fig. S1c–e ). Figure 1: Distribution of Gβ2 protein on the surface of mitochondria. ( a ) Immunostaining with a specific antibody shows the localization of Gβ2 in HeLa cells. Cells were stained with 20 nM Mitotracker Red, and then immuno-labelled with anti-Gβ2 (green) and visualized with a two-photon microscope (Zeiss, LSM 510). The boxed area on the upper left was scanned along the Z axis, and the images were superposed to form the three-dimensional (3D) image. The boxed area in the 3D image is shown at higher magnification in the upper right panels. The lower right shows images of Y to Z dimension. Scale bar, 20 μm. ( b ) Distribution of Gβ1, Gα12, Gαi1 and Gγ2 in HeLa cells. Representative images of HeLa cells labelled with anti-Gβ1, Gα12, Gαi1 and Gγ2 antibodies (green) and stained with 20 nM Mitotracker Red. Scale bar, 10 μm. ( c ) Distribution of Gβ2 and other G proteins in the mitochondrial fraction. Equal amounts of the whole cell lysate (W), cytosol (C 1 ), light membrane (C 2 ), mitochondria (M) and plasma membrane (P) fractions were loaded and analysed for the distribution of Gβ2, Gγ2 and other G proteins by western blot using specific antibodies. The purity of isolated mitochondria was determined by using the markers for distinct organelles: Mfn1, VDAC1 (mitochondria), GM130 (Golgi), p62 (endoplasmic reticulum) and actin (cytoplasm). ( d ) Protease K assay for Gβ2's localization on mitochondria. Mitochondrial fractionation obtained from HeLa cells was subjected to Protease K digestion for 30 min with different concentrations as indicated. Gβ2 and other mitochondrial proteins such as Mfn1, Tom20 (outer mitochondrial membrane, OMM) and Tim23 (inner mitochondrial membrane, IMM) were analysed by western blot with corresponding antibodies. Equal amounts of protein were loaded for Protease K treatment. ( e ) Gβ2 is the most abundant subunit of Gβ proteins in HeLa cells. mRNA levels of distinct Gβ subunits were analysed by semiquantitative PCR in HeLa cells. ( f , g ) The mRNA levels of Gα, Gγ subunits in the cells were analysed by semiquantitative PCR (right panel). The size markers are 1,000, 750, 500, 200 and 100 bp, respectively, from top to bottom. All the experiments were repeated at least three times. Full size image Gβ2 physically interacts with Mfn1 We next determined whether there is indeed a physical interaction between Gβ2 and Mfn1. Endogenous Gβ2 was coimmunoprecipitated with Mfn1 but not with normal mouse immunoglobulin-G from HeLa cell lysate. Importantly, depletion of Gβ2 in the cells by short hairpin RNA (shRNA) abolished the interaction, whereas Gβ2 could be co-immunoprecipitated with Mfn1 after Gβ2 was reintroduced into the shRNA cells, and vice versa, when Mfn1 was used as the bait ( Fig. 2a,b ). However, we failed to detect an interaction between Gβ2 and Mfn2, Gβ2 and Drp1, or Gβ1 and Mfn1 ( Supplementary Fig. S2a–c ) or between Gβ2 and Gα12, which is reportedly localized in mitochondria [24] . There was a weak interaction of Gβ2 with Gαi1, although the significance of this interaction remains to be determined. To validate our findings that Gβ2 interacted directly with Mfn1, we performed two independent fluorescence resonance energy transfer (FRET) analyses on HeLa cells co-transfected with Mfn1-CFP and Gβ2-YFP. In the cells, the expressed Mfn1-CFP was specifically localized in mitochondria, whereas a majority of YFP-Gβ2 was found in mitochondria ( Supplementary Fig. S2d ). In this assay, the fluorescent intensity of the donor CFP was measured before and after the fluorescence of the acceptor YFP was photobleached (quenched). 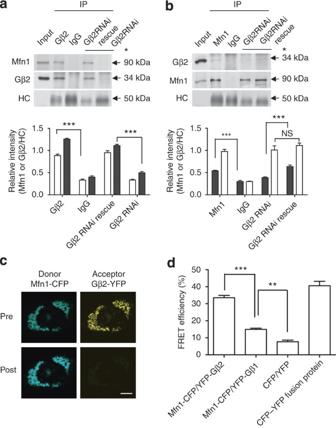Figure 2: Gβ2 physically interacts with Mfn1 to induce mitochondrial aggregation. (a) Immunoprecipitation (IP) of Gβ2 with Mfn1. Lysates either from HeLa cells, or cells expressing a shRNA specific to Gβ2 or the latter reintroduced with a mutant of Flag-Gβ2 carrying a mutation for eliminating the RNAi target sequence (the right two lanes marked as asterisk), were incubated with a Gβ2 antibody overnight, followed by western blot with an anti-Mfn1 antibody. The crude lysates from these cells were used as input. (b) Mfn1 coimmunoprecipitates with Gβ2. The cell lysates were incubated with Mfn1 antibody overnight, followed by western blot with an anti-Gβ2 antibody. Mfn1, Gβ2 and heavy chain (HC) levels were quantified by densitomery. Relative intensity were obtained as intensity of bands of Mfn1 (opened box) or Gβ2 (filled box) divided by intensity of heavy chain of relative lines. Error bars represent the s.e.m.,n=3; *** forP<0.0005, two-tailed test. (c) Images of fluorescence intensity from the cells co-transfected with CFP-Mfn1 and YFP-Gβ2 in CFP and YFP channels before and after photobleaching of YFP. The increase of the CFP fluorescence and dramatic decrease of the YFP fluorescence were observed after the photobleaching, Scale bar, 10 μm. (d) The histogram shows the FRET efficiency from CFP to YFP in the cells transfected with both CFP-Mfn1 and YFP-Gβ2, CFP-Mfn1 and YFP-Gβ1, CFP–YFP fusion protein and both of CFP and YFP, respectively. Error bars represent the s.e.m.,n=18; Differences in the mean FRET efficiency between CFP-Mfn1 and YFP-Gβ2, CFP-Mfn1 and YFP-Gβ1, or CFP and YFP were statistically significant at ***P<0.0005, **P<0.005, two-tailedt-test. As shown in Figure 2c , the fluorescent intensity of CFP was remarkably increased after the fluorescence of YFP was completely quenched by a laser beam. This observation suggested that there was a direct interaction between Mfn1-CFP and Gβ2-YFP in the cells. The energy transfer efficiency from CFP to YFP obtained by using the equation described [26] was 33.9%. In contrast, energy transfer efficiency from Mfn1-CFP to Gβ1-YFP was significantly lower (only ~10%) ( Fig. 2d ). Taken together, our data demonstrate that Mfn1 and Gβ2 have a physical interaction and that the interaction is specific. We next determined the structural domains responsible for the interaction of Gβ2 and Mfn1. Co-immunoprecipitation of truncated mutants of Mfn1 and Flag-tagged Gβ2 in HeLa cells revealed that, consistent with the yeast two hybrid assay, the domain of Mfn1 from aa241 to 350 was necessary for the interaction between Mfn1 and Gβ2 ( Fig. 3a,b ). Also, the Mfn1 mutant lacking the interaction domain had diminished FRET ( Supplementary Fig. S2e ). Importantly, we found that Mfn1 lacking the interacting domain from aa241–350 failed to induce mitochondrial aggregation compared with that of wild-type Mfn1 ( Fig. 3c ), whereas GTPase dead mutants Mfn1 T109A and K88T were able to induce mitochondrial aggregation ( Supplementary Fig. S2f ). Our results thus identify that, in addition to the heptad repeat region (HR2) domain of Mfn1 [15] , the domain between the GTPase domain and the HR1 domain is also important for mitochondrial fusion by its interaction with Gβ2. On the other hand, we generated a series of Flag-tagged Gβ2 with various truncations of WD repeats and transfected these constructs into HeLa cells ( Fig. 3d ), and found that they failed to induce mitochondrial aggregation ( Fig. 3e ). Co-immunoprecipitation revealed that the deletion of four WD40 repeats of Gβ2 completely abolished its interaction with Mfn1 ( Fig. 3f ), suggesting that the toroidal structure needs to be intact for their interaction and subsequent mitochondrial fusion. Figure 2: Gβ2 physically interacts with Mfn1 to induce mitochondrial aggregation. ( a ) Immunoprecipitation (IP) of Gβ2 with Mfn1. Lysates either from HeLa cells, or cells expressing a shRNA specific to Gβ2 or the latter reintroduced with a mutant of Flag-Gβ2 carrying a mutation for eliminating the RNAi target sequence (the right two lanes marked as asterisk), were incubated with a Gβ2 antibody overnight, followed by western blot with an anti-Mfn1 antibody. The crude lysates from these cells were used as input. ( b ) Mfn1 coimmunoprecipitates with Gβ2. The cell lysates were incubated with Mfn1 antibody overnight, followed by western blot with an anti-Gβ2 antibody. Mfn1, Gβ2 and heavy chain (HC) levels were quantified by densitomery. Relative intensity were obtained as intensity of bands of Mfn1 (opened box) or Gβ2 (filled box) divided by intensity of heavy chain of relative lines. Error bars represent the s.e.m., n =3; *** for P <0.0005, two-tailed test. ( c ) Images of fluorescence intensity from the cells co-transfected with CFP-Mfn1 and YFP-Gβ2 in CFP and YFP channels before and after photobleaching of YFP. The increase of the CFP fluorescence and dramatic decrease of the YFP fluorescence were observed after the photobleaching, Scale bar, 10 μm. ( d ) The histogram shows the FRET efficiency from CFP to YFP in the cells transfected with both CFP-Mfn1 and YFP-Gβ2, CFP-Mfn1 and YFP-Gβ1, CFP–YFP fusion protein and both of CFP and YFP, respectively. Error bars represent the s.e.m., n =18; Differences in the mean FRET efficiency between CFP-Mfn1 and YFP-Gβ2, CFP-Mfn1 and YFP-Gβ1, or CFP and YFP were statistically significant at *** P <0.0005, ** P <0.005, two-tailed t -test. 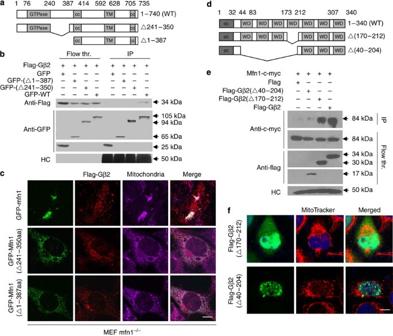Figure 3: Identification of the interacting domain between Mfn1 and Gβ2. (a) GTPase domain (aa 76–240), two coiled-coil domains (aa 387–414 and 705–735), and transmembrane domain (aa592–628) are indicated as filled grey boxes. A mutant lacking aa 241–350 was named as Δ241–350; the Δ1–387 construct contains only C-terminal amino acids from 387 to 740. (b) Cell lysates from the HeLa cells expressing Flag-Gβ2 with either GFP-Mfn1 or GFP- Mfn1 (Δ241–350) or GFP-Mfn1 (Δ1–387) or GFP as indicated were subjected to immunoprecipitation with an antibody against GFP, followed by western blot with a Flag antibody. The heavy chain of immunoglobulins was used as loading control. (c) The confocal images of Mfn1−/−MEFs expressing the Flag-Gβ2 (Red) with either GFP- Mfn1 or GFP-Mfn1 (Δ241–350) or GFP-Mfn1 (Δ1–387), and mitchondria are visualized with Mitotracker deep red. Scale bar, 10 μm. (d) Coiled-coil domain (aa1–32) and seven WD40 domains (aa 44–83, 86–125, 132–170, 173–212, 215–254, 257–298 and 307–340) are indicated as filled grey boxes. The mutants lacking the fourth or the first four WD40 domains were named as Δ171–212 and Δ40–204, respectively. (e) Lysates either from HeLa cells co-transfected mfn1-c-myc with Flag-Gβ2, Flag-Gβ2 (Δ171–212), Flag-Gβ2 (Δ40–204) or Flag as indicated were subjected to IP with an antibody against Flag, followed by western blots with a c-myc antibody. (f) The representative images of the HeLa cells expressing the Flag-Gβ2 (Δ171–212) or Flag- Gβ2 (Δ40–204) (green) and mitochondria were visualized with 20 nM MitoTracker Red. Full size image Figure 3: Identification of the interacting domain between Mfn1 and Gβ2. ( a ) GTPase domain (aa 76–240), two coiled-coil domains (aa 387–414 and 705–735), and transmembrane domain (aa592–628) are indicated as filled grey boxes. A mutant lacking aa 241–350 was named as Δ241–350; the Δ1–387 construct contains only C-terminal amino acids from 387 to 740. ( b ) Cell lysates from the HeLa cells expressing Flag-Gβ2 with either GFP-Mfn1 or GFP- Mfn1 (Δ241–350) or GFP-Mfn1 (Δ1–387) or GFP as indicated were subjected to immunoprecipitation with an antibody against GFP, followed by western blot with a Flag antibody. The heavy chain of immunoglobulins was used as loading control. ( c ) The confocal images of Mfn1 −/− MEFs expressing the Flag-Gβ2 (Red) with either GFP- Mfn1 or GFP-Mfn1 (Δ241–350) or GFP-Mfn1 (Δ1–387), and mitchondria are visualized with Mitotracker deep red. Scale bar, 10 μm. ( d ) Coiled-coil domain (aa1–32) and seven WD40 domains (aa 44–83, 86–125, 132–170, 173–212, 215–254, 257–298 and 307–340) are indicated as filled grey boxes. The mutants lacking the fourth or the first four WD40 domains were named as Δ171–212 and Δ40–204, respectively. ( e ) Lysates either from HeLa cells co-transfected mfn1-c-myc with Flag-Gβ2, Flag-Gβ2 (Δ171–212), Flag-Gβ2 (Δ40–204) or Flag as indicated were subjected to IP with an antibody against Flag, followed by western blots with a c-myc antibody. ( f ) The representative images of the HeLa cells expressing the Flag-Gβ2 (Δ171–212) or Flag- Gβ2 (Δ40–204) (green) and mitochondria were visualized with 20 nM MitoTracker Red. Full size image Gβ2 requires Mfn1 for its effect on mitochondrial dynamics We then addressed the biological significance of the interaction between Gβ2 and Mfn1. 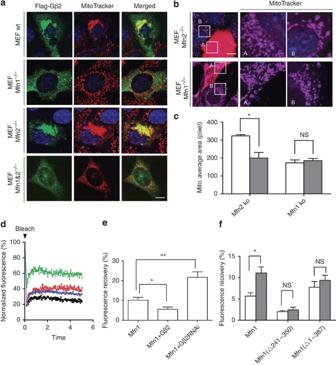Figure 4: Gβ2 requires Mfn1 for its effect on mitochondrial dynamics. (a) Representative images of wild type or Mfn1−/−and/or Mfn2−/−MEF cells transfected with Flag-tagged Gβ2. Mitochondria in cells were stained with MitoTracker Red and Flag- Gβ2 were immunostained with a Flag-specific antibody. Scale bar, 10 μm. (b) Mitochondria in Mfn2−/−cells, and Mfn1−/−cells are shown in the representative images of Mfn1−/−or Mfn2−/−MEFs transfected with Gβ2 shRNA (red). The box area A (tranfected cell) and B (untransfectd cell) in the left panel show the different mitochondrial size at higher magnifications. Scale bar, 10 μm. (c) The quantification of mitochondrial size scored by Image J (Wayne Rasband, NIH). Filled box represents mitochondrial size in Mfn2−/−MEFs and open box represents in Mfn2−/−MEFs transfected with Gβ2 shRNA. The data represent the mean s.d.,n=10–15. Differences in the mean mitochondrial average area between mfn2−/−MEFs and mfn2−/−MEFs with Gβ2 shRNA were statistically significant at *P<0.05. (d) Mfn1-YFP was co-transfected into HeLa cells with either Flag- Gβ2 (, black) or Gβ2 shRNA (, red) and the mitochondrial Mfn1 mobility was measured by FRAP. Fis1 (, green) was used as a control of fast membrane mobility as previously reported28and Mfn1 alone (, blue) was used as baseline control. Each line represents the mean of ≥20 measurements. (e) The fluorescence recovery of Mfn1-YFP in HeLa cells and the cells co-transfected with either Flag-Gβ2 or Gβ2 shRNA was measured by FRAP. Differences in the mean fluorescence recovery between Mfn1-YFP in HeLa cells and Mfn1-YFP in HeLa cells co-transfected with Flag-Gβ2, or with Gβ2 shRNA were statistically significant *P<0.05 and **P<0.005; Error bars represent the s.e.m.,n=21. (f) Mobility of Mfn1-GFP, or Mfn1-GFP (Δ241–350), Mfn1-GFP (Δ1–387) in HeLa cells and the cells co-transfected with DsRed-Gβ2 shRNA was measured by FRAP. The fluorescence recovery of Mfn1-GFP, Mfn1-GFP (Δ241–350) and Mfn1-GFP (Δ1–387) in HeLa cells and the cells co-transfected with Gβ2 shRNA was measured by FRAP. *P<0.05 and NS means nonsignificant. Data represent the mean s.e.m.,n=20. As shown in Figure 4a , Gβ2 induced mitochondrial aggregation in both wild-type and Mfn2 −/− MEF cells, in which Mfn1 is expressed. However, ectopic expression of Gβ2 failed to induce mitochondrial aggregation in Mfn1 −/− cells (Mfn1 −/− or Mfn1&2 −/− MEF cells). These data support our notion that Gβ2 indeed requires Mfn1 for regulating mitochondrial fusion. A previous study has shown [27] that mitochondria are spheres or ovals and maintain a certain degree of fusion in Mfn2 −/− MEF cells compared with that of Mfn1 −/− MEF cells. Interestingly, Gβ2 shRNA could further fragment mitochondria, resulting in the size of mitochondria similar to that in Mfn1 −/− MEFs. In contrast, it had little effect on the mitochondrial morphology in Mfn1 −/− MEF cells ( Fig. 4b,c ). It is also interesting to note that Gβ2 localizes at the specific submitochondrial locations where mitochondria appear to have the tendency of branching along mitochondrial tubular structure (see Fig. 1a ). Collectively, these data suggest that Gβ2 regulates the mitochondrial fusion, which requires Mfn1. Figure 4: Gβ2 requires Mfn1 for its effect on mitochondrial dynamics. ( a ) Representative images of wild type or Mfn1 −/− and/or Mfn2 −/− MEF cells transfected with Flag-tagged Gβ2. Mitochondria in cells were stained with MitoTracker Red and Flag- Gβ2 were immunostained with a Flag-specific antibody. Scale bar, 10 μm. ( b ) Mitochondria in Mfn2 −/− cells, and Mfn1 −/− cells are shown in the representative images of Mfn1 −/− or Mfn2 −/− MEFs transfected with Gβ2 shRNA (red). The box area A (tranfected cell) and B (untransfectd cell) in the left panel show the different mitochondrial size at higher magnifications. Scale bar, 10 μm. ( c ) The quantification of mitochondrial size scored by Image J (Wayne Rasband, NIH). Filled box represents mitochondrial size in Mfn2 −/− MEFs and open box represents in Mfn2 −/− MEFs transfected with Gβ2 shRNA. The data represent the mean s.d., n =10–15. Differences in the mean mitochondrial average area between mfn2 −/− MEFs and mfn2 −/− MEFs with Gβ2 shRNA were statistically significant at * P <0.05. ( d ) Mfn1-YFP was co-transfected into HeLa cells with either Flag- Gβ2 ( , black) or Gβ2 shRNA ( , red) and the mitochondrial Mfn1 mobility was measured by FRAP. Fis1 ( , green) was used as a control of fast membrane mobility as previously reported [28] and Mfn1 alone ( , blue) was used as baseline control. Each line represents the mean of ≥20 measurements. ( e ) The fluorescence recovery of Mfn1-YFP in HeLa cells and the cells co-transfected with either Flag-Gβ2 or Gβ2 shRNA was measured by FRAP. Differences in the mean fluorescence recovery between Mfn1-YFP in HeLa cells and Mfn1-YFP in HeLa cells co-transfected with Flag-Gβ2, or with Gβ2 shRNA were statistically significant * P <0.05 and ** P <0.005; Error bars represent the s.e.m., n =21. ( f ) Mobility of Mfn1-GFP, or Mfn1-GFP (Δ241–350), Mfn1-GFP (Δ1–387) in HeLa cells and the cells co-transfected with DsRed-Gβ2 shRNA was measured by FRAP. The fluorescence recovery of Mfn1-GFP, Mfn1-GFP (Δ241–350) and Mfn1-GFP (Δ1–387) in HeLa cells and the cells co-transfected with Gβ2 shRNA was measured by FRAP. * P <0.05 and NS means nonsignificant. Data represent the mean s.e.m., n =20. Full size image Gβ2 regulates the mobility of Mfn1 on the mitochondria It is possible that Gβ2 regulates mitochondrial fusion by affecting the distribution of Mfn1 on the microregion of mitochondrial surface and thereby the membrane mobility of Mfn1. To test this hypothesis, we measured the Mfn1 membrane mobility in the presence or absence of Gβ2 using a FRAP assay. This technique provides a semiquantitative measurement of the movement of the mitochondrial proteins by assessing the depth of bleaching and rate of redistribution of mitochondrial outer membrane-localized yellow/green fluorescence protein (Mfn1-YFP was used in the assay ( Supplementary Fig. S3a )) into regions of irreversible fluorophore photobleach [28] . Intriguingly, downregulation of Gβ2 by shRNA in HeLa cells caused an increase of Mfn1 mobility, whereas overexpression of Gβ2 caused a significant decrease in the mobility of Mfn1 ( Fig. 4d,e ). In addition, Gβ2 shRNA failed to increase the mobility of Mfn1 mutants (Δ241–350 and Δ1–387) that lack the interacting domain ( Fig. 4f ). This finding further supports our notion that their interaction is critical for the mobility of Mfn1 on the outer membrane surface of mitochondria. In contrast, the mobility of Mfn2 showed little change when Gβ2 was downregulated in HeLa cells ( Supplementary Fig. S3b,c ). Moreover, it was evidenced that Gβ2 failed to localize at the mitochondria in MEF Mfn1 −/− cells ( Supplementary Fig. S3d ) unless Mfn1 was reintroduced into these cells (J.Z., unpublished observation). A fractionation assay further showed that Gβ2 levels were significantly reduced in Mfn1 −/− cells ( Supplementary Fig. S3e ). These observations suggest that the interaction between Gβ2 and Mfn1 may help to regulate their submitochondrial distribution and the mobility of Mfn1, which may be important for determining the fusion or branching at particular submitochondrial regions. Depletion of Gβ2 decreases mitochondrial fusion To determine whether endogenous Gβ2 has a regulatory function in mitochondrial fusion, we used Gβ2 shRNA to deplete endogenous Gβ2 ( Supplementary Fig. S4a ). Interestingly, loss of Gβ2 resulted in a notable change in mitochondrial networking as indicated by mito-green fluorescent protein (GFP) labelling. The mitochondria became small tubules and spheres around the nuclear region, most likely due to impaired mitochondrial fusion ( Fig. 5a ). The effect of Gβ2 on mitochondria was specific, as reintroduction of Gβ2 into these cells significantly rescued the mitochondrial phenotypes ( Fig. 5b,c ). Mitochondrial dynamics was analysed by using an assay of visualization and quantification of mitochondrial fusion, based on confocal imaging of cells expressing a mitochondrial matrix-targeted photoactivable GFP (PAGFP) dilution rate [29] . Compared with the fast decrease of mito-PAGFP fluorescence intensity of activated mitochondria in normal HeLa cells observed 30 min after photoactivation, little change or no decrease in mito-PAGFP fluorescence within photoactivated mitochondria in HeLa cells with Gβ2 shRNA was seen ( Fig. 5d–f ), reflecting slower mitochondrial fusion rate. The result thus indicates that mitochondrial fusion was blocked by Gβ2 shRNA. In addition, overexpression of Flag-Gβ2 significantly caused aggregation of mitochondria around the nucleus in HeLa ( Supplementary Fig. S4b , upper panel) and SH-SY5Y cells (not shown), as revealed by confocal microscopy. To further determine that Gβ2 in mitochondria regulates mitochondrial fusion, we constructed mitochondrial targeted Gβ2 using a specific mitochondrial outer membrane targeting signal peptide from Bcl-xL [30] . Overexpression of mitochondrial targeted Gβ2 induced profound mitochondrial aggregation at the perinuclear region in HeLa cells. In contrast, mitochondrial targeted Gγ2 or GFP protein using the same mitochondrial targeting signal had no effect on mitochondrial morphology ( Supplementary Fig. S4b , middle and lower panel). Electron microscopy analysis further confirmed that the mitochondria clustered and aggregated around the perinuclear region when Gβ2 was ectopically expressed ( Supplementary Fig. S4c ). 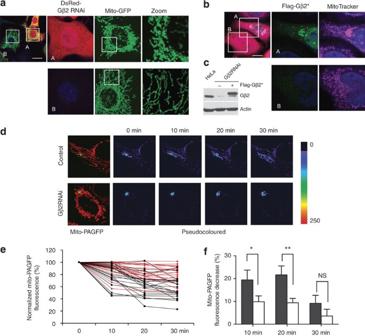Figure 5: Gβ2 has a regulatory role in mitochondrial morphology. (a) HeLa cells were co-transfected with DsRed-Gβ2 shRNA (red) and mitochondrial matrix localized GFP (mito-GFP), and the expression of Gβ2 shRNA (box A) and mitochondrial morphology was visualized by confocal microscopy (left panel). Scale bar, 10 μm. (b) Gβ2 shRNA HeLa cells (red) were transfected with a mutant of Flag-Gβ2 (green) as described inFigure 2. The cells were stained with 10 nM Mitotracker Deep Red for visualizing mitochondria. Scale bar, 10 μm. (c) The Gβ2 protein levels in the cells were determined by western blot: HeLa cells (left lane), HeLa cells with either Gβ2 shRNA (middle lane) or Gβ2 shRNA with reintroduced mutant of Flag-Gβ2 (right lane). (d) Gβ2 RNAi block mitochondrial fusion. HeLa cells and Gβ2 shRNA stable cells were transfected with mito-PAGFP and followed by photoactivation. Images were collected every 10 min over 30 min. Representative images shown are pseudo-coloured projections of z-series to represent changes in the fluorescence intensities. The fluorescence intensity of mito-PAGFP is highlighted in the pseudocoloured images where fusion of photoactivated 'orange' mitochondria with nonactivated 'purple' organelles is followed by the formation of the 'yellow/blue' intermediates. (e) Normalized fluorescence intensity of mito-PAGFP in HeLa cells (black) and Gβ2 shRNA stable cells (red) at each time point was measured and plotted against time. Each experimental group contains at least 20 cells. (f) Values of percent mito-PAGFP fluorescence in HeLa cells and Gβ2 shRNA stable cells decrease after 10, 20, and 30 min in each experimental group, and were plotted against time. Filled box represents Gβ2 shRNA cells and open box represents normal HeLa cells. The error bars represent s.e.m.,n=26 cell time-lapse measurements per group. Differences in the mean fluorescence decrease percentage between HeLa cells and HeLa cells with Gβ2 shRNA in 10 min and in 20 min were statistically significant *P<0.05 and **P<0.005, two-tailedt-test. Figure 5: Gβ2 has a regulatory role in mitochondrial morphology. ( a ) HeLa cells were co-transfected with DsRed-Gβ2 shRNA (red) and mitochondrial matrix localized GFP (mito-GFP), and the expression of Gβ2 shRNA (box A) and mitochondrial morphology was visualized by confocal microscopy (left panel). Scale bar, 10 μm. ( b ) Gβ2 shRNA HeLa cells (red) were transfected with a mutant of Flag-Gβ2 (green) as described in Figure 2 . The cells were stained with 10 nM Mitotracker Deep Red for visualizing mitochondria. Scale bar, 10 μm. ( c ) The Gβ2 protein levels in the cells were determined by western blot: HeLa cells (left lane), HeLa cells with either Gβ2 shRNA (middle lane) or Gβ2 shRNA with reintroduced mutant of Flag-Gβ2 (right lane). ( d ) Gβ2 RNAi block mitochondrial fusion. HeLa cells and Gβ2 shRNA stable cells were transfected with mito-PAGFP and followed by photoactivation. Images were collected every 10 min over 30 min. Representative images shown are pseudo-coloured projections of z-series to represent changes in the fluorescence intensities. The fluorescence intensity of mito-PAGFP is highlighted in the pseudocoloured images where fusion of photoactivated 'orange' mitochondria with nonactivated 'purple' organelles is followed by the formation of the 'yellow/blue' intermediates. ( e ) Normalized fluorescence intensity of mito-PAGFP in HeLa cells (black) and Gβ2 shRNA stable cells (red) at each time point was measured and plotted against time. Each experimental group contains at least 20 cells. ( f ) Values of percent mito-PAGFP fluorescence in HeLa cells and Gβ2 shRNA stable cells decrease after 10, 20, and 30 min in each experimental group, and were plotted against time. Filled box represents Gβ2 shRNA cells and open box represents normal HeLa cells. The error bars represent s.e.m., n =26 cell time-lapse measurements per group. Differences in the mean fluorescence decrease percentage between HeLa cells and HeLa cells with Gβ2 shRNA in 10 min and in 20 min were statistically significant * P <0.05 and ** P <0.005, two-tailed t -test. Full size image The effects of Gβ2 on mitochondria are specific We next determined if the effects of Gβ2 on mitochondria are specific. Overexpression of Gβ2 had little impact on the morphology and distribution of other cellular organelles such as Golgi, lysosomes or endoplasmic reticulum in HeLa cells ( Fig. 6a ). To determine the effect of Gβ2 on mitochondrial physiology and function, we measured mitochondrial membrane potential in the HeLa cells overexpressing Gβ2 by using TMRM (tetramethylrhodamine, methyl ester) staining and found that there was no significant difference from the parental cells (see Supplementary Fig. S4d ). Furthermore, Gβ2 did not seem to have any effect on the cell cycle (see Supplementary Fig. S4e,f ). 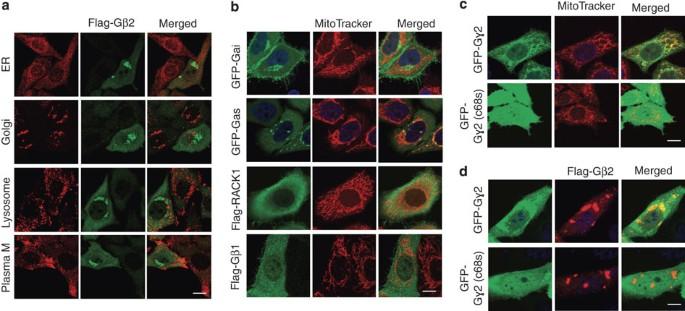Figure 6: The effects of Gβ2 on mitochondria are specific. (a) Representative images of morphology of endoplasmic reticulum, lysosomes, Golgi, plasma membrane in HeLa cells with enforced expression of Flag-Gβ2. HeLa cells were transfected with Flag-Gβ2. After incubation for 24 h, the cells were fixed in 4% paraformadehyde and double immunostained Flag (green) with either of the antibodies: Calnexin, GM130, Lamp3 or Transferrin receptor (red). (b) HeLa cells were transiently transfected with GFP- Gαi1, GFP-Gαs, Flag-tagged Gβ1or Flag-tagged RACK1, respectively. The cells were then loaded with 20 nM MitoTracker Red for visualizing mitochondria, and immunostained Flag (green) for labelling Flag-tagged Gβ1or Flag-tagged RACK1. (c) Confocal images of HeLa cells transfected with GFP-Gγ2 or Gγ2 (C68S). After incubation for 24 h, the cells were stained with Mitotracker (red). (d) HeLa cells co-transfected Flag-Gβ2 with GFP-Gγ2 or Gγ2 (C68S), and the cell were fixed and immunostained with Flag antibody (red). Sale bar, 10 μm. Figure 6: The effects of Gβ2 on mitochondria are specific. ( a ) Representative images of morphology of endoplasmic reticulum, lysosomes, Golgi, plasma membrane in HeLa cells with enforced expression of Flag-Gβ2. HeLa cells were transfected with Flag-Gβ2. After incubation for 24 h, the cells were fixed in 4% paraformadehyde and double immunostained Flag (green) with either of the antibodies: Calnexin, GM130, Lamp3 or Transferrin receptor (red). ( b ) HeLa cells were transiently transfected with GFP- Gαi1, GFP-Gαs, Flag-tagged Gβ1or Flag-tagged RACK1, respectively. The cells were then loaded with 20 nM MitoTracker Red for visualizing mitochondria, and immunostained Flag (green) for labelling Flag-tagged Gβ1or Flag-tagged RACK1. ( c ) Confocal images of HeLa cells transfected with GFP-Gγ2 or Gγ2 (C68S). After incubation for 24 h, the cells were stained with Mitotracker (red). ( d ) HeLa cells co-transfected Flag-Gβ2 with GFP-Gγ2 or Gγ2 (C68S), and the cell were fixed and immunostained with Flag antibody (red). Sale bar, 10 μm. Full size image The surprising finding that Gβ2 has such a regulatory role in controlling mitochondrial fusion prompted us to test if other Gβ subunits and Gα or Gγ also have a role in mitochondria. We found that Gβ1 induced a small fraction (10%) of cells with mitochondrial aggregation, whereas other Gβ proteins failed to alter mitochondrial morphology ( Fig. 6b ). RACK1, a protein also named Gβ2-like protein 1 with WD40 repeat domains, could not induce mitochondrial aggregation in the cells ( Fig. 6b ). Gγ2 or its mutant form (C68S), which fails to localize at the membrane, did neither affect mitochondrial morphology nor the distribution of Gβ2 ( Fig. 6c,d ). Ectopic expression of Gα proteins, such as Gαi1 or Gαs, failed to induce the alteration of mitochondrial morphology or restore dysfunctioned network of mitochondria induced by Gβ2 knockdown ( Fig. 7a ). Mitochondrial aggregation was evident when cells were co-transfected with Gβ2 and Gγ2, or Gβ2 plus Gαil and Gγ2 ( Fig. 7a,b ), although the overall percentage of transfected cells with aggregated mitochondria was slightly reduced compared with that in cells expressing Gβ2 alone or Gβ2 together with Gαi1 ( Fig. 7c ). Gβ2 lacking the Gγ interacting domain is still able to induce the mitochondrial aggregation; even when it is coexpressed with Gγ2. Moreover, ectopic expression of Gγ2 failed to restore fragmented mitochondria induced by Gβ2 knockdown ( Fig. 7d–f ). Taken together, we demonstrate that the effect of Gβ2 on mitochondria is unique and Gγ2 has limited effect on the regulatory role of Gβ2 on mitochondrial fusion. 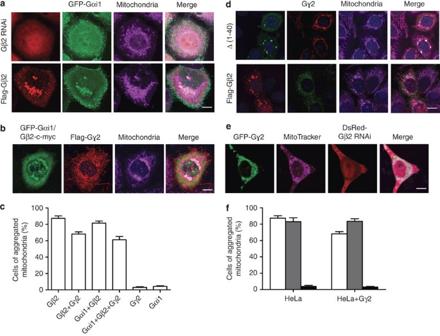Figure 7: Gαi1 and Gγ2 proteins have limited effects on Gβ2-induced mitochondrial aggregation. (a) Upper panels: Gβ2 shRNA HeLa cells (red) were transfected with GFP-Gαi1 (green) and loaded with 20 nM MitoTracker Deep Red; bottom panels: HeLa cells were co-transfected with GFP-Gαi1 and Flag-Gβ2 (red) and loaded with 20 nM MitoTracker Deep Red. (b) HeLa cells were transfected with Flag-Gγ2, Gβ2-c-myc and YFP-Gαi1. After incubation for 24 h, the cells were incubated with Mitotracker (Deep Red), fixed and immunostained with Flag antibody (red) and c-myc antibody (green). (c) The histogram indicates the mitochondrial aggregation percentage in the cells transfected with either of the coupled pairs: Flag-Gβ2 alone, Flag-Gβ2 and Gγ2, Flag-Gβ2, Gγ2 and YFP-Gαi1, Flag-Gβ2 and YFP-Gαi1, YFP-Gαi1 alone and Gγ2 alone, respectively. Overall, 350–400 cells were counted in each experiment. Error bars represent the s.e.m. (d) HeLa cells were transfected with Gγ2 and Flag-Gβ2 or Flag-Gβ2 (Δ1–40). After incubation for 24 h, the cells were incubated with Mitotracker (Deep Red), fixed and immunostained with Flag antibody and Gγ2 antibody. (e) Gβ2 shRNA HeLa cells (red) were transfected with Flag-Gγ2 (green) and loaded with 20 nM MitoTracker Deep Red. The scale bar in all images represents 10 μm. (f) The histogram indicates the mitochondrial aggregation percentage in the cells transfected with either of the coupled pairs: Flag-Gβ2 alone (open box), Flag-Gβ2 (Δ1–40) (grey box), Flag-Gβ2 and Gγ2 (open box), Flag-Gβ2 (Δ1–40) and Gγ2 (grey box), Gγ2 alone and null vector (filled box), respectively. Error bars represent the s.e.m. Quantification was carried out as described inc. Figure 7: Gαi1 and Gγ2 proteins have limited effects on Gβ2-induced mitochondrial aggregation. ( a ) Upper panels: Gβ2 shRNA HeLa cells (red) were transfected with GFP-Gαi1 (green) and loaded with 20 nM MitoTracker Deep Red; bottom panels: HeLa cells were co-transfected with GFP-Gαi1 and Flag-Gβ2 (red) and loaded with 20 nM MitoTracker Deep Red. ( b ) HeLa cells were transfected with Flag-Gγ2, Gβ2-c-myc and YFP-Gαi1. After incubation for 24 h, the cells were incubated with Mitotracker (Deep Red), fixed and immunostained with Flag antibody (red) and c-myc antibody (green). ( c ) The histogram indicates the mitochondrial aggregation percentage in the cells transfected with either of the coupled pairs: Flag-Gβ2 alone, Flag-Gβ2 and Gγ2, Flag-Gβ2, Gγ2 and YFP-Gαi1, Flag-Gβ2 and YFP-Gαi1, YFP-Gαi1 alone and Gγ2 alone, respectively. Overall, 350–400 cells were counted in each experiment. Error bars represent the s.e.m. ( d ) HeLa cells were transfected with Gγ2 and Flag-Gβ2 or Flag-Gβ2 (Δ1–40). After incubation for 24 h, the cells were incubated with Mitotracker (Deep Red), fixed and immunostained with Flag antibody and Gγ2 antibody. ( e ) Gβ2 shRNA HeLa cells (red) were transfected with Flag-Gγ2 (green) and loaded with 20 nM MitoTracker Deep Red. The scale bar in all images represents 10 μm. ( f ) The histogram indicates the mitochondrial aggregation percentage in the cells transfected with either of the coupled pairs: Flag-Gβ2 alone (open box), Flag-Gβ2 (Δ1–40) (grey box), Flag-Gβ2 and Gγ2 (open box), Flag-Gβ2 (Δ1–40) and Gγ2 (grey box), Gγ2 alone and null vector (filled box), respectively. Error bars represent the s.e.m. Quantification was carried out as described in c . Full size image Our results have demonstrated a novel role of Gβ2 in Mfn1-dependent mitochondrial fusion. We found that mitochondrial Gβ2 interacts with Mfn1 and regulates the mobility of Mfn1. It is possible that Gβ2, as a scaffold protein [31] , may function to mediate the clustering of Mfn1 molecules at the microregion of the mitochondrial outer membrane. As a result, Gβ2 may modulate the distribution and activity of Mfn1, which could be important in mitochondrial fusion or branching at specific submitochondrial sites. Intriguingly, several WD40 proteins were found to interact with Dnm1 (Drp1 homologue in yeast), a key protein in mediating fission, for mitochondrial fission [13] , [32] and Caf4 regulates the polarized distribution of Dnm1 [12] . Thus, it is of great interest to note that distinct proteins with WD40 repeat domains are involved in both mitochondrial fusion and fission by regulating the submitochondrial distribution of proteins for these processes. On the plasma membrane, Gβγ interacts with Gα and subsequently transduces signals to the downstream effectors. We found that G-protein-coupled receptor activators (ET1, PGE2) or antagonists (PTX), which are known to affect the dissociation/association of Gα and Gβγ, did not have any effect on mitochondrial networking or Gβ2-induced changes in mitochondrial networking (J.Z., unpublished observations). These data do not support that the activation of G-protein-coupled receptor signalling pathway or the translocation of Gβγ from the plasma membrane onto mitochondria are important for the altered mitochondrial networking observed. The combinatorial expression of Gαi1 and Gγ2 proteins has limited effects on Gβ2-induced mitochondrial aggregation (see Fig. 7 ). Mutant Gγ2-C68S, which fails to be modified by lipid and fails to localize to mitochondria, also did not affect mitochondrial morphology induced by enforced expression of Gβ2. Recently, it has been reported that Gα12 and Gαi1 are found to localize on the surface of mitochondria [23] , [24] . However, their role in mitochondria is largely unknown. We detected a weak interaction between Gβ2 with Gαi, but not with Gα12, although both are found in mitochondria. More studies are needed to further dissect the significant role of G proteins in regulating mitochondrial phenotypes and the interplay between mitochondria and other cellular events. Previous studies have also shown that Gβγ interacts with dynein and tubulin [33] to regulate microtubule reorganization and cell polarity [18] , [19] . Indeed, we have found that Gβ2 was able to interact with tubulin in co-immunoprecipitation analysis (data not shown). A Gβ protein was also found to interact with dynein intermediate chain, a member in the dynein family [31] . The interaction of Gβ2 with microtubules or motor proteins may provide an additional force for bringing mitochondria in proximity for mitochondrial tethering and docking, leading to an initiation of fusion. Plasmid construction and mutagenesis The human Mfn1 cDNA obtained from Dr Margaret Fuller (Stanford University, USA) was subcloned into a plasmid vector pECFP-N1 (Clontech) using Eco RI and Bam HI. The Gβ2 gene was cloned by PCR from a human fetal liver cDNA library, and the Gβ2 cDNA was inserted into plasmid vectors pFLAG-CMV-4 (Sigma) and pEYFP-C1 (Clontech) to generate pFLAG-Gβ2 and pEYFP-Gβ2 using Hin dIII and Eco RI, respectively. The cDNA fragment encoding the Bcl-xL mitochondrial target peptide was amplified by PCR and fused to the C terminal of Gβ2 in pFLAG-Gβ2, named as Flag-Gβ2-M. The GFP 10 -GNG2 and pEGFP-GNB1 plasmids were from Dr Terence E. Hébert (McGill University, Canada). The Gγ2 cDNA was subcloned to pFLAG-CMV-4 and the mutant (C68S) of GFP 10 -Gγ2 was generated by site-directed mutagenesis. Flag-Gγ2-M was generated as described above. The GNB1 cDNA was subcloned to pEYFP-C1 and pFLAG-CMV-4 using Hin dIII and Kpn I, respectively. The cDNA fragment encoding the mitochondrial matrix-localized signal peptide of TRX2 was subcloned to pEYFP-C1 and pEGFP-C1 using Eco RI and Bam HI. The QuickChange site-directed mutagenesis kit was purchased from Stratagene. The GNB2 RNAi target sequences: CCTGGATGACAACCAAATC were designed by company (RuiBo) and subcloned to the RNAi-Ready pSIREN-RetroQ-DsRed-Express Vector (Clontech). Antibodies and reagents Antibodies to Gβ1, Gβ2, Gγ2, Gα12, Gαi1, RACK1, c-Myc, VDAC1 and LAMP3 were purchased from Santa Cruz, and the concentrations of them are 200 μg ml −1 . Antibodies to Flag and α-tubulin were from Sigma, and the concentrations of both are 1 mg ml −1 . Antibodies to Tom20, Tim23, GM130, Transferrin receptor and Calnexin were from Becton Dickinson, and the concentrations of them are 1 mg ml −1 . Antibodies to Mfn1 and Mfn2 monoclonal were from Novus, the concentrations of both are 500 μg ml −1 . The antibodies were diluted 1:100 of the original concentration for immunostaining and diluted 1:1,000–1:5,000 for western blotting. Mitotracker Red and Mitotracker Deep Red were purchased from Invitrogen. Cell culture and transfections Mfn1 and Mfn2 knockout, and Mfn1 and Mfn2 double knockout MEF cells were kind gifts from Dr David Chan (California Institute of Technology). HeLa and SH-SY5Y cells (American Type Culture Collection) were maintained in Dulbecco's modified Eagle's medium with 10% fetal bovine serum, 100 U ml −1 penicillin and 100 U ml −1 streptomycin at 37 °C in a 5% CO 2 incubator. Cells were transfected with plasmid DNAs by using a phosphate calcium method. Confocal microscopy HeLa and SH-SY5Y cells cultured on gelatin-coated coverslips were fixed with 3.7% paraformaldehyde, followed by permeabilization in 0.5% Triton X-100. Cells were incubated with primary antibodies in phosphate-buffered saline (PBS) supplemented with 5% bovine serum albumin, followed by incubation with appropriate secondary antibodies. To visualize mitochondria in living cells, cells were incubated with either MitoTracker Deep Red 633 or Red CMXRos (Invitrogen) at 37 °C for 30 min and washed twice with PBS. Images were visualized under an LSM 510 confocal microscope (Carl Zeiss), equipped with 63×/1.45 oil objective and processed using LSM Browser (Carl Zeiss) and Photoshop (Adobe). Mitochondria fractionation The mitochondrial membrane was purified on discontinuous sucrose gradients as previously described [34] , with some modifications. Briefly, cells were washed twice in PBS and resuspended in 1.5 ml buffer A (20 mM Tricine, 250 mM sucrose) containing protease inhibitors for 20 min on ice and then subjected to homogenization. After 20 strokes, the cell homogenate was collected and 100 μl of the samples were taken out as whole cell lysate (W). The remaining cell homogenate was centrifuged at 1,000× g for 8 min at 4 °C, and the supernatant was as the postnuclear solution (PNS). PNS (100 μl) was centrifuged at 10,000× g , and the supernant was collected as C2. PNS (2 ml) was layered on a Percoll gradient (30%) and centrifuged at 30,000× g for 30 min at 4 °C, a white band (1–2 ml) at 2 cm in Percoll gradient just below the PNS was collected as the plasma membrane fraction (P). P was continuingly centrifuged at 100,000× g for 1 h at 4 °C to remove the percoll. Another PNS (2 ml) was centrifuged at 10,000× g , and the pellet was washed twice with Buffer B (0.225 M mannitol, 1 mM EGTA, 25 mM HEPES, pH 7.4) and resuspended in 0.5 ml Buffer B. The suspension was layered to a Percoll density gradient (2 ml 80%, 4.5 ml 52% and 4.25 ml 26%) and centrifuged at 100,000× g for 1 h at 4 °C. The band between the Percoll 26% and 52% gradient was collected as the pure mitochondrial fractionation (M). C1 was the supernatant obtained after the cell homogenate was centrifuged at 250,000× g for 1 h at 4 °C. Mitochondria membrane motility assay The mitochondria membrane motility was measured as previous described [28] . Briefly, circular region of interests (ROIs), 2.5 mm in diameter, were imaged (a-Plan-FLUAR 100×/1.45 oil objective; Carl Zeiss) before and after photobleaching (20 iterations of 514-nm laser (488-nm laser for GFP) set to 100%) of 0.5-mm circular ROIs located in the centre of imaging area. Totally, 150 images (1 scan every 33 ms) were collected and the fluorescence intensity was digitalized in imaged ROIs with an LSM 510 software (Zeiss MicroImaging). FRET assay All FRET observations were performed under a Leica DM IRE2 confocal laser scanning microscope, after cells were transfected for 24 h. The donor (CFP) was excited at 458 nm, and its fluorescence was detected in a wavelength of 478–498 nm (CFP channel), whereas the excitation at 514 nm and the emission at 545±15 nm were used for detecting the acceptor (YFP) (YFP channel). FRET was detected at the excitation of 458 nm and the emission of 545±15 nm (FRET channel). Fluorescence images of the transfected cells were taken at the CFP-, YFP- and FRET channels sequentially. Dequenching of the donor fluorescence by photobleaching of the acceptor YFP was performed by illuminating the transfected cells at the YFP excitation wavelength (514 nm) for 250 iterations, and then the CFP-Mfn1 images were taken at the same focal plane. The FRET efficiency was calculated using the equation: E =1−( F DA / F D ), where F DA and F D are the fluorescence intensity of CFP in the cells expressing both donor and acceptor, and donor alone (acceptor was quenched), respectively [26] . Immunoprecipitation Cells were collected and washed twice with PBS, and then resuspended in lysis buffer (0.75 M aminocaproic acid, 50 mM Bis-Tris, pH 7.0, 1.5% n -dodecyl-b-d-maltopyranoside, 1 mM phenylmethyl sulphonyl fluoride, 1 mg ml −1 leutpeptin and 1 mg ml −1 pepstatin) for 30 min on ice, and, then subjected to centrifugation at 72,000 g for 20 min at 4 °C. The primary monoclonal antibody (2 μg) was added into the supernatant containing 500 μg proteins, and incubated at 4 °C overnight. After incubation with Protein G-agarose (Santa Cruz Biotech) for 2 h at 4 °C, the beads were washed three times with the lysis buffer and boiled with 6× loading buffer for 5 min. The proteins were then separated by SDS–polyacrylamide gel electrophoresis, and western blotting was performed with proper antibodies as indicated. Mitochondrial membrane potential assay The mitochondrial membrane potential was measured. Briefly, HeLa cells were transfected with an empty vector and pFlag-Gβ2. After 24 h, the cells were collected and stained with 200 nM TMRM (Invitrogen) for 15 min at room temperature, and then kept at 4 °C for measurement after washing once with PBS. For each sample, 50,000 cells were scored after excitation with a 488 nm argon laser and emission through the phycoerythrin filter (575 nm) of a flow cytometer (Becton Dickinson). The percentile of cells above and below the threshold TMRM fluorescence signal was determined with Cellquest software. Cell cycle analysis Cells were collected and washed and then resuspended in PBS. The cell suspension containing 1×10 6 cells in 500 μl was fixed by adding 5 ml cold (−20 °C) 75% ethanol at 4 °C overnight. The cells were centrifuged at 1,000× g for 10 min at 4 °C and washed twice with 5 ml PBS plus 1% bovine serum albumin, and resuspended in 400 μl PBS supplemented with 1% bovine serum albumin, 50 μl 500 μg ml −1 propidium iodide and 50 μl boiled RNase A (10 mg ml −1 ). After incubating at 37 °C for 30 min, the cells were analysed by FACS using an FL2 histogram at 620 nm (Becton Dickinson). Photoactivation assay Cells were grown in two-well chambers for confocal microscopy. Images were captured with a microscope (model LSM 510; Carl Zeiss MicroImaging) using a 63×1.4 NA Apochromat objective (Carl Zeiss MicroImaging). Light (405- or 413-nm) was used for photoactivation of PAGFP. ROIs were selected and series of z-sections from the top to the cell bottom with intervals between sections set to 0.5–0.75 μm were irradiated with 405- or 413-nm light. The same intervals between optical sections were used for imaging. How to cite this article: Zhang, J. et al . G-protein β2 subunit interacts with mitofusin 1 to regulate mitochondrial fusion. Nat. Commun. 1:101 doi: 10.1038/ncomms1099 (2010).